A closed-loop synthetic gene circuit for the treatment of diet-induced obesity in mice Diet-induced obesity is a lifestyle-associated medical condition that increases the risk of developing cardiovascular disease, type 2 diabetes and certain types of cancer. Here we report the design of a closed-loop genetic circuit that constantly monitors blood fatty acid levels in the setting of diet-associated hyperlipidemia and coordinates reversible and adjustable expression of the clinically licensed appetite-suppressing peptide hormone pramlintide. Grafting of the peroxisome proliferator-activated receptor-α onto the phloretin-responsive repressor TtgR produces a synthetic intracellular lipid-sensing receptor (LSR) that reversibly induces chimeric TtgR-specific promoters in a fatty acid-adjustable manner. Mice with diet-induced obesity in which microencapsulated cells engineered for LSR-driven expression of pramlintide are implanted show significant reduction in food consumption, blood lipid levels and body weight when put on a high-fat diet. Therapeutic designer circuits that monitor levels of pathologic metabolites and link these with the tailored expression of protein pharmaceuticals may provide new opportunities for the treatment of metabolic disorders. Diet-induced obesity typically results from a combination of excessive food energy intake, favoured by an evolutionary remain associating energy-dense food with greater taste, lack of physical activity and genetic susceptibility [1] . Obesity is at the origin of a wide range of diseases such as cardiovascular disorders, type 2 diabetes, obstructive sleep apnea, osteoarthritis, asthma and certain types of cancer, and has become a leading preventable cause of death with dramatically increasing prevalence, affecting up to 1.5 billion people in industrialized and developing countries [2] , [3] , [4] . A sustainable change in lifestyle, including dieting and physical exercise, is the pillar for the treatment of obesity that can be complemented by gastric balloon and bariatric surgery to assist weight loss [4] and by taking anti-obesity drugs to reduce appetite or fat absorption [5] , [6] , [7] . However, dieting often shows limited success [8] , surgery is associated with significant risks [9] and only some anti-obesity drugs with modest efficacy [10] remain on the market after many have been withdrawn because of side effects [11] , [12] , [13] , [14] , and few have entered clinical trials since [15] . The amylin analogue pramlintide has recently been licensed as injection-based adjunctive type 2 diabetes therapy [16] , as it reduces adsorption of glucose and other nutrients such as fat by slowing gastric emptying, promotes satiety via GLP-1-independent hypothalamic receptors and inhibits inappropriate secretion of glucagon [17] . However, precise injection-based dosing at mealtime remains challenging [18] . Synthetic biology-inspired designer networks that coordinate caloric intake to satiety responses could control dietary energy homeostasis and may provide a new strategy for the treatment of obesity. In humans, peroxisome proliferator-activated receptor-α (PPARα) is a nuclear lipid receptor heterodimerizing with the retinoic X receptor to form a transcription factor that constitutively binds to specific target promoters [19] , [20] . Through interaction with regulatory co-activators such as the steroid receptor coactivator 1 (ref. 21 ), the PPAR-γ coactivator 1 (ref. 22 ), the CREB-binding protein (CBP) [22] and the E1A binding protein p300 (ref. 22 ) or with specific co-repressors like the nuclear receptor corepressor (NCoR) [23] , [24] , [25] , the G-protein pathway suppressor 2 (GPS2) [26] and the histone deacetylase (HDAC3) [26] PPARα manages uptake, utilization and catabolism of fatty acids in a variety of tissues such as the liver, kidney, heart, muscle and adipose. PPARα’s activity is modulated by binding of fatty acids [27] , [28] (for example, linoleic acid, a plant-derived fatty acid and palmitic acid, an animal-derived fatty acid) and synthetic fibrate drugs licensed for the treatment of hyperlipidemia [29] . In this study we take advantage of PPARα’s capacity to detect a variety of fatty acids to score diet-dependent blood fat levels and to correct diet-induced obesity in mice by expressing a clinically licensed appetite-suppressing peptide hormone. Closed-loop synthetic gene networks operating inside vascularized designer-cell implants that constantly monitor circulating disease-relevant metabolites, process off-level concentrations and coordinate production and release of a specific protein therapeutic in a self-sufficient manner may become a treatment strategy of the future. Design of a synthetic mammalian lipid-sensing receptor We have fused the ligand-binding domain of PPARα to the bacterial DNA-binding repressor TtgR [30] to create a binary synthetic transcription factor, the lipid-sensing receptor (LSR), which retains dual-input sensitivity to fatty acids (via PPARα) as well as to the transdermal cosmetic additive phloretin [31] (via TtgR), and specifically binds (via TtgR) and modulates (via PPARα) transcription of chimeric promoters (P TtgR1 ) in an adjustable manner ( Fig. 1a ). Whereas LSR’s PPARα domain recruits co-repressors (NCoR, GPS2 and HDAC3) in the absence of fatty acids, which silence P TtgR1 -driven transgene expression ( Fig. 1a,b ), they become replaced by co-activators (PPAR-γ coactivator 1, CBP, steroid receptor coactivator 1 and p300) on binding of lipids, which activates P TtgR1 -mediated transcription in a dose-dependent manner. Lipid-dependent modulation of P TtgR1 exclusively occurs when LSR is bound to the promoter via its TtgR domain in the absence of phloretin, whereas in the presence of this trigger compound, LSR is released from P TtgR1 and transcription shut down irrespective of the lipid status of the cells. Thus, LSR’s TtgR domain ensures promoter specificity and provides a potential trigger-inducible safety switch to override lipid-dependent promoter activation ( Fig. 1a ). Cotransfection of several rodent, primate and human cell lines with the constitutive LSR expression vector pKR135 (P hCMV -LSR-pA; LSR, TtgR-PPARα) and the LSR-dependent secreted alkaline phosphatase (SEAP) reporter construct pMG10 (ref. 30 ; P TtgR1 -SEAP-pA) showed that SEAP was exclusively and dose-dependently induced whenever the cells were exposed to exogenous linoleic acid ( Fig. 1c ). As the isogenic transcription factor TtgA 1 (pMG11 (ref. 30 ), TtgR-VP16) was insensitive to fatty acids in an identical experimental set-up, LSR’s lipid-sensing capacity indeed resides in its PPARα domain while the TtgR moiety mediates sequence-specific binding ( Supplementary Fig. S1a ). Differences in the cellular portfolio of promiscuous PPARα-coregulatory components and lipid metabolism may in part explain the differences in basal expression and induction profiles among different cell lines ( Fig. 1c ). Control experiments showed that neither ectopic expression of LSR (SEAP level: +LSR (pKR135/pSEAP2-Control), 87.9±2.7 U l −1 ; −LSR (pcDNA3.1/pSEAP2-Control), 87.4±6.9 U l −1 ) nor exposure of the cells to excessive fatty acid concentrations had a negative impact on their viability ( Supplementary Fig. S1b ). In addition, specificity and leakiness tests confirmed that LSR’s target promoter P TtgR1 was neither induced by endogenous components nor activated by unrelated synthetic transcription factors ( Supplementary Fig. S2a ). Further experiments using different constitutive promoters to drive LSR and different LSR-specific target promoters confirmed that the combination of pKR135, pMG10 and HT-1080 cells showed the best fatty acid-triggered transgene induction and was therefore used in all follow-up experiments ( Fig. 1d,e ). 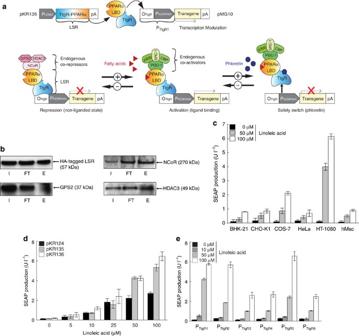Figure 1: A synthetic fatty acid-responsive mammalian gene switch. (a) The synthetic lipid-controlled mammalian transcription device consists of an intracellular LSR, a fusion protein combining the phloretin-responsive repressor (TtgR) and the human PPARα, which binds a TtgR-specific operator (OTtgR) linked to a minimal promoter (PhCMVmin) (PTtgR1) to control transgene expression. In the absence of fatty acids, LSR associates with an inhibitory complex (GPS2, G-protein pathway suppressor 2; HDAC, histone deacetylase; NCoR, nuclear receptor corepressor) to repress transgene expression, which switches to full induction in the presence of fatty acids when LSR associates with the activation complex (SRC1, steroid receptor coactivator 1; p300, E1A binding protein; CBP, CREB-binding protein; PGC-1, peroxisome proliferator-activated receptor-γ coactivator). Transgene expression can also be shut down by disrupting LSR-promoter binding by addition of the clinically licensed skin-penetrating apple metabolite phloretin. (b) Co-immunoprecipitation. HT-1080 were cotransfected with pKR151 (encoding HA-tagged LSR) and pMG10, and the co-repressors (NCoR, GPS2 and HDAC3) interacting with LSR were identified by protein complex CoIP after 48 h. E, eluate; FT, flow through; I, input. (c) Linoleic acid-induced SEAP expression in different cell lines. Cells were co-transfected with the LSR-encoding expression vector (pKR135; PhCMV-LSR-pA) and the PTtgR1-driven SEAP expression plasmid (pMG10; PhCMV*-1-SEAP-pA), grown in the presence of different linoleic acid concentrations, and SEAP levels were profiled in the culture supernatant after 48 h. (d,e) Optimization of the LSR’s fatty acid sensitivity. (d) HT-1080 were (co-)transfected with pMG10 (PTtgR1-SEAP-pA) and an expression vector encoding LSR under control of different constitutive promoters (pKR124, PSV40-LSR-pA; pKR135, PhCMV-LSR-pA; pKR136, PhEF1α-LSR-pA) and cultivated in the presence of increasing concentrations of linoleic acid for 48 h before SEAP was profiled in the culture supernatant. (e) HT-1080 were (co-)transfected with the LSR expression vector pKR135 (PhCMV-LSR-pA) and reporter constructs encoding SEAP under control of different LSR-specific promoter variants containing 0 (PTtgR1; pMG10 (ref.30)), 2 (PTtgR2; pMG20 (ref.30)), 4 (PTtgR3; pMG21 (ref.30)), 6 (PTtgR4; pMG22 (ref.30)), 8 (PTtgR5; pMG23 (ref.30)) and 10 (PTtgR6; pMG24 (ref.30)) base pair linkers between the TtgR operator (OTtgR) and the minimal promoter (PhCMVmin). Transfected HT-1080 were cultivated in the presence of different linoleic acid concentrations and SEAP expression was profiled after 48 h. Error bars indicate s.d. (n=4). Figure 1: A synthetic fatty acid-responsive mammalian gene switch. ( a ) The synthetic lipid-controlled mammalian transcription device consists of an intracellular LSR, a fusion protein combining the phloretin-responsive repressor (TtgR) and the human PPARα, which binds a TtgR-specific operator (O TtgR ) linked to a minimal promoter (P hCMVmin ) (P TtgR1 ) to control transgene expression. In the absence of fatty acids, LSR associates with an inhibitory complex (GPS2, G-protein pathway suppressor 2; HDAC, histone deacetylase; NCoR, nuclear receptor corepressor) to repress transgene expression, which switches to full induction in the presence of fatty acids when LSR associates with the activation complex (SRC1, steroid receptor coactivator 1; p300, E1A binding protein; CBP, CREB-binding protein; PGC-1, peroxisome proliferator-activated receptor-γ coactivator). Transgene expression can also be shut down by disrupting LSR-promoter binding by addition of the clinically licensed skin-penetrating apple metabolite phloretin. ( b ) Co-immunoprecipitation. HT-1080 were cotransfected with pKR151 (encoding HA-tagged LSR) and pMG10, and the co-repressors (NCoR, GPS2 and HDAC3) interacting with LSR were identified by protein complex CoIP after 48 h. E, eluate; FT, flow through; I, input. ( c ) Linoleic acid-induced SEAP expression in different cell lines. Cells were co-transfected with the LSR-encoding expression vector (pKR135; P hCMV -LSR-pA) and the P TtgR1 -driven SEAP expression plasmid (pMG10; P hCMV*-1 -SEAP-pA), grown in the presence of different linoleic acid concentrations, and SEAP levels were profiled in the culture supernatant after 48 h. ( d , e ) Optimization of the LSR’s fatty acid sensitivity. ( d ) HT-1080 were (co-)transfected with pMG10 (P TtgR1 -SEAP-pA) and an expression vector encoding LSR under control of different constitutive promoters (pKR124, P SV40 -LSR-pA; pKR135, P hCMV -LSR-pA; pKR136, P hEF1α -LSR-pA) and cultivated in the presence of increasing concentrations of linoleic acid for 48 h before SEAP was profiled in the culture supernatant. ( e ) HT-1080 were (co-)transfected with the LSR expression vector pKR135 (P hCMV -LSR-pA) and reporter constructs encoding SEAP under control of different LSR-specific promoter variants containing 0 (P TtgR1 ; pMG10 (ref. 30 )), 2 (P TtgR2 ; pMG20 (ref. 30 )), 4 (P TtgR3 ; pMG21 (ref. 30 )), 6 (P TtgR4 ; pMG22 (ref. 30 )), 8 (P TtgR5 ; pMG23 (ref. 30 )) and 10 (P TtgR6 ; pMG24 (ref. 30 )) base pair linkers between the TtgR operator (O TtgR ) and the minimal promoter (P hCMVmin ). Transfected HT-1080 were cultivated in the presence of different linoleic acid concentrations and SEAP expression was profiled after 48 h. Error bars indicate s.d. ( n =4). Full size image LSR characterization and control by fatty acids and fibrates Detailed characterization of pKR135/pMG10-transgenic HT-1080 cells revealed that the synthetic fatty acid sensor circuit was fully reversible ( Fig. 2a ) and precisely adjusted transgene expression levels in response to a wide range of fatty acid concentrations ( Fig. 2b ). At the same time, LSR retained its dose-dependent sensitivity to the licensed cosmetic additive phloretin [32] that could release LSR from P TtgR1 , override fatty acid-induced transcription control and shut down transgene expression ( Fig. 2c ). 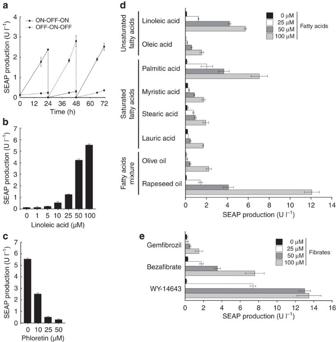Figure 2: Characterization of fatty acid-controlled transgene expression. (a) Reversibility of fatty acid-responsive SEAP expression was assessed by cultivating transgenic HT-1080 (pKR135/pMG10) for 72 h while alternating the linoleic acid status of the culture (100 μM ON, 0 μM OFF) at 24 and 48 h. (b) Adjustability of fatty-acid-inducible SEAP expression. pKR135-/pMG10-transgenic HT-1080 were cultivated in medium containing increasing linoleic acid concentrations and corresponding SEAP production was quantified in the culture supernatant after 48 h. (c) Phloretin-triggered safety switch. pKR135-/pMG10-engineered HT-1080 were programmed for maximum expression by 100 μM linoleic acid followed by addition of different concentrations of phloretin before SEAP expression was scored after 48 h. (d) Sensitivity of the LSR control switch to different fatty acids. HT-1080 containing the LSR device were exposed for 48 h to different concentrations of specific fatty acids before SEAP expression was assessed. (e) Tunability of the LSR control device in response to clinically licensed fibrate drugs. LSR-transgenic HT-1080 (pKR135/pMG10) were cultivated in the presence of different concentrations of fibrate drugs and SEAP production was profiled after 48 h. Error bars indicate s.d. (n=3). Figure 2: Characterization of fatty acid-controlled transgene expression. ( a ) Reversibility of fatty acid-responsive SEAP expression was assessed by cultivating transgenic HT-1080 (pKR135/pMG10) for 72 h while alternating the linoleic acid status of the culture (100 μM ON, 0 μM OFF) at 24 and 48 h. ( b ) Adjustability of fatty-acid-inducible SEAP expression. pKR135-/pMG10-transgenic HT-1080 were cultivated in medium containing increasing linoleic acid concentrations and corresponding SEAP production was quantified in the culture supernatant after 48 h. ( c ) Phloretin-triggered safety switch. pKR135-/pMG10-engineered HT-1080 were programmed for maximum expression by 100 μM linoleic acid followed by addition of different concentrations of phloretin before SEAP expression was scored after 48 h. ( d ) Sensitivity of the LSR control switch to different fatty acids. HT-1080 containing the LSR device were exposed for 48 h to different concentrations of specific fatty acids before SEAP expression was assessed. ( e ) Tunability of the LSR control device in response to clinically licensed fibrate drugs. LSR-transgenic HT-1080 (pKR135/pMG10) were cultivated in the presence of different concentrations of fibrate drugs and SEAP production was profiled after 48 h. Error bars indicate s.d. ( n =3). Full size image Interestingly, LSR was sensitive to a broad spectrum of fatty acids, including unsaturated (linoleic acid and oleic acid) and saturated (palmitic acid, myristic acid, stearic acid and lauric acid) ones of plant (linoleic acid) and animal (palmitic acid, stearic acid and myristic acid) origin, as well as to complex fatty acids mixtures such as dietary oils ( Fig. 2d ). For example, although linoleic and palmitic acids mediated up to 55-fold induction of SEAP expression, rapeseed oil reached induction factors of up to 140 ( Fig. 2d ). LSR is also sensitive to fibrates such as WY-14643, gemfibrozil (LOPID) and bezafibrate (BEZALIP) ( Fig. 2e ), a class of synthetic amphipathic carboxylic acids that are clinically licensed for the treatment of hyperlipidemia [29] . This suggests that the LSR controller device could also be used for drug-controlled expression of therapeutic transgenes and combined with fibrate-based therapies. Fatty acid-mediated transgene expression in mice Covering a wide range of dietary and synthetic fatty acids at high sensitivity, the LSR-based sensor device has all its takes to precisely score physiologic fatty acid levels. To validate fatty acid-triggered product gene expression in vivo , pKR135/pMG10-transgenic HT-1080 variants engineered for fatty acid-controlled SEAP expression were microencapsulated in coherent alginate-poly-( l -lysine)-alginate beads [33] , which is the preferred cell implant material known for its optimal pore-size tunability [34] , metabolic and immuno-isolation [34] and vascularization [35] , [36] , as well as for long-term support of cell functionality [34] , [35] , [36] , [37] , [38] and low inflammatory reaction [36] . The microencapsulated circuit-transgenic cells were implanted into the peritoneal cavity of wild-type mice kept on a standard diet. Previous studies have shown that intraperitoneally implanted alginate-encapsulated cells become vascularized and connected to the bloodstream [36] , and that fatty acids reach a rapid diffusion-based equilibrium between the the peritoneal cavity and the peripheral circulation [39] . The animals were treated with diverse concentrations of linoleic and palmitic acid, or received different oral doses of rapeseed oil, whereas control mice obtained an identical fatty acid-free care. Mice with LSR implants that were treated with lipid supplements showed a significant dose-dependent increase of SEAP in their serum ( Fig. 3a,b ). This suggests that the LSR sensor device was able to monitor, process and report hyperlipidemia in vivo , whereas the circuit remains shut down at physiologic blood fat levels reached during a standard diet. To confirm the in-vivo precision of the LSR sensor device, we also implanted microencapsulated pKR135/pMG10-transgenic HT-1080 cells into diet-induced obese mice put on medium-fat (MF; 10 kcal% fat) and high-fat (HF; 60 kcal% fat) diets, and compared their blood fatty acid and SEAP levels to non-obese control animals with a standard caloric low-fat intake (LF; 5 kcal% fat; Fig. 3c,d ). LSR-transgenic cell implants were able to indirectly score the food quality by sensing specific blood fat levels represented by serum cholesterol and phospholipids [40] , [41] , [42] , [43] ( Fig. 3c ) and produced the corresponding SEAP expression response that resulted in serum SEAP levels specific for each diet group ( Fig. 3d ). Control animals receiving isogenic pMG10 (P TtgR1 -SEAP-pA)-containing implants lacking LSR had no detectable SEAP circulating in their bloodstream ( Supplementary Fig. S2b ). 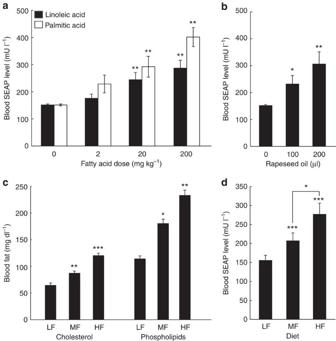Figure 3: Performance of fatty acid-inducible expression control in wild-type mice. (a–d) Standard low fat-fed wild-type mice were implanted with per microencapsulated pKR135-/pMG10-transgenic HT-1080 (2 × 106cells per mouse) and received different doses of linoleic/palmitic acids (a), rapeseed oil (b) or were put on standard LF, (5 kcal% fat), MF (10 kcal% fat) and HF (60 kcal% fat) diets (c,d). Resulting blood SEAP levels (a,b,d) and blood fat levels represented by serum cholesterol and phospholipid concentrations (c) were quantified after 48 h (a,b,d) or 72 h (c). Data are mean ±s.e.m., statistics by two-tailed Student’st-test;n=8 mice per group. *P<0.05, **P<0.005, ***P<0.0001 versus zero lipid doses (a,b) or LF mice (c,d). Figure 3: Performance of fatty acid-inducible expression control in wild-type mice. ( a – d ) Standard low fat-fed wild-type mice were implanted with per microencapsulated pKR135-/pMG10-transgenic HT-1080 (2 × 10 6 cells per mouse) and received different doses of linoleic/palmitic acids ( a ), rapeseed oil ( b ) or were put on standard LF, (5 kcal% fat), MF (10 kcal% fat) and HF (60 kcal% fat) diets ( c , d ). Resulting blood SEAP levels ( a , b , d ) and blood fat levels represented by serum cholesterol and phospholipid concentrations ( c ) were quantified after 48 h ( a , b , d ) or 72 h ( c ). Data are mean ±s.e.m., statistics by two-tailed Student’s t -test; n =8 mice per group. * P <0.05, ** P <0.005, *** P <0.0001 versus zero lipid doses ( a , b ) or LF mice ( c , d ). Full size image Application of LSR in diet-induced obese mice To automatically control diet-induced obesity in a self-sufficient manner, we functionally coupled the LSR sensor device to expression of the clinically licensed anorectic peptide hormone pramlintide [7] , which suppresses appetite, promotes satiety [5] and slows gastric emptying [44] , thereby limiting high-caloric food intake, attenuating hyperlipidemic blood levels, reducing body weight and restoring the energy homeostasis of the organism. Therefore, we replaced SEAP of pMG10 by pramlintide and validated the resulting vector pK146 (P TtgR1 -Pram-pA) for LSR-controlled pramlintide production using enzyme-linked immunosoebent assay (ELISA; Supplementary Fig. S3a ) as well as a cell-based assay, confirming pramlintide’s capacity to activate its target CALC/RAMP receptor and trigger the corresponding signalling cascades ( Supplementary Fig. S3b ). To test the designer circuit’s capacity to control diet-induced obesity, we implanted pKR135/pKR146-engineered HT-1080 into diet-induced obese mice receiving HF (60 kcal% fat) or MF (10 kcal% fat) diets, as well as wild-type mice receiving standard food (LF; 5 kcal% fat) and profiled pramlintide levels, blood fat concentrations, food intake and body weight for several days ( Fig. 4 ). Although treated diet-induced obese mice showed a significant diet-dependent increase in circulating pramlintide levels ( Fig. 4a ) leading to reduction of blood fat levels ( Fig. 4b ), food consumption ( Fig. 4c ) and body weight ( Fig. 4d ), all of these values remained unchanged in control animals receiving standard food ( Fig. 4a–d ). In addition, pramlintide levels in the plasma of animals receiving isogenic LSR-free but pKR146 (P TtgR1 -Pram-pA)-containing control implants were almost undetectable ( Supplementary Fig. S2c ). It is of particular importance that standard-fed wild-type mice implanted with the LSR-driven pramlintide device kept their body weight, suggesting that the designer network is only active in an obesity-risk situation involving excess fat and stops pramlintide production to prevent underfeeding ( Fig. 4a,d ). Visual analysis of the capsules in the peritoneal cavity ( Fig. 4e ) and profiling of the inflammatory indicators interleukin-6 (IL-6) and tumour necrosis factor-α (TNF-α) in treated animals of different diet groups (LF, MF and HF diets) showed no detectable inflammation ( Supplementary Fig. S4 ). 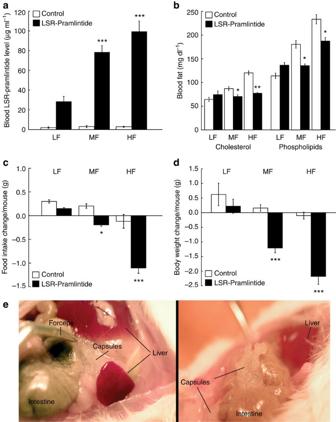Figure 4: Self-sufficient LSR-based control of pramlintide expression in diet-induced obese mice. (a–d) Mice fed for 14 weeks with standard LF (5 kcal% fat), MF (10 kcal% fat) and HF (60 kcal% fat) diets were implanted with pKR135/pKR146-transgenic HT-1080 (2 × 106cells per mouse) (LSR-Pramlintide) or the isogenic pKR135/pMG10-transgenic HT-1080 (2 × 106cells per mouse) (Control). Seventy-two hours after implantation, blood pramlintide levels (a) and blood fat levels represented by serum cholesterol and phospholipid concentrations (b), as well as change in food intake (c) and weight loss (d) were profiled. (e) Illustrations showing implanted microencapsulated circuit-transgenic HT-1080 (pKR135/pKR146) of two different dissected mice. Data are mean±s.e.m., statistics by two-tailed Student’st-test;n=8 mice per group. *P<0.05, **P<0.005, ***P<0.0001 versus LF mice. Figure 4: Self-sufficient LSR-based control of pramlintide expression in diet-induced obese mice. ( a – d ) Mice fed for 14 weeks with standard LF (5 kcal% fat), MF (10 kcal% fat) and HF (60 kcal% fat) diets were implanted with pKR135/pKR146-transgenic HT-1080 (2 × 10 6 cells per mouse) (LSR-Pramlintide) or the isogenic pKR135/pMG10-transgenic HT-1080 (2 × 10 6 cells per mouse) (Control). Seventy-two hours after implantation, blood pramlintide levels ( a ) and blood fat levels represented by serum cholesterol and phospholipid concentrations ( b ), as well as change in food intake ( c ) and weight loss ( d ) were profiled. ( e ) Illustrations showing implanted microencapsulated circuit-transgenic HT-1080 (pKR135/pKR146) of two different dissected mice. Data are mean±s.e.m., statistics by two-tailed Student’s t -test; n =8 mice per group. * P <0.05, ** P <0.005, *** P <0.0001 versus LF mice. Full size image Synthetic biology-inspired control devices and gene networks that precisely reprogram the dynamic behaviour, metabolism and physiology of mammalian cells have reached a level of sophistication [45] , which enables the community to rapidly move forward and start to shape new clinical applications and treatment concepts [46] , [47] , [48] . Therapeutic networks combining sensor and effector devices that, on integration into cells and functional connection to their metabolism, monitor disease-relevant metabolites, process on/off level control and coordinate adjusted therapeutic responses that restore metabolite homeostasis in a seamless, automatic and self-sufficient manner are particularly attractive for future gene and cell-based therapies. The closed-loop LSR-pramlintide circuit represents a prototype for such a therapeutic designer circuit. The LSR sensor captures a wide range of lipids within their physiologic concentration range, becomes dose-dependently activated by peak fatty acid levels and shuts down at native concentrations. In combination with the pramlintide-encoding effector component and implanted into diet-induced obese mice, the designer circuit (i) constantly monitored blood fatty acid levels, (ii) processed peak fat values, (iii) produced a coordinated pramlintide production response that (iv) reduced food intake, (v) decreased blood fat levels, (vi) dropped the body weight and (vii) automatically switched off at normal blood fat levels.In addition, as the LSR used TtgR as a DNA-binding component the designer device can be switched off at any time using a skin lotion containing the clinically licensed apple metabolite phloretin [32] , which may represent an additional safety latch in future clinical applications. With obesity being on its way to develop into a global epidemic, available pharmacotherapies showing limited success and an almost dried-out drug pipeline [14] , [15] , [16] , [17] , [18] synthetic biology-inspired cell-based therapies may foster new opportunities in the treatment of obesity and related metabolic diseases. It is now conceivable that autologous designer cells that are implanted into humans inside vascularizing semi-permeable microcontainers monitor disease-relevant metabolites in the peripheral circulation and coordinate expression of relevant therapeutic proteins in an emerging pathologic situation [36] , [38] , [49] , [50] . As designer cell implants are scalable to the patients’ needs could be replaced by ambulant interventions and removed in acute situations or after completion of therapy, they may become a pillar in future personalized medicine programmes [51] , [52] . Lipid sensor components Comprehensive design and construction details for all expression vectors are provided in Supplementary Table S1 . Key plasmids include the following: pKR135 encoding constitutive expression of the LSR (P hCMV -LSR-pA); pMG10 (ref. 30 ) harbouring a SEAP expression unit driven by the LSR-specific phloretin-responsive promoter (P TtgR1 ; P TtgR1 -SEAP-pA); and pKR146 containing a P TtgR1 -driven pramlintide expression unit (P TtgR1 -Pram-pA). Cell culture and transfection Human embryonic kidney cells (HEK-293T, ATCC: CRL-11268), Baby hamster kidney cells (BHK-21, ATCC: CCL-10), African green monkey kidney cells (COS-7, ATCC: CRL-1651), human cervical adenocarcinoma cells (HeLa, ATCC: CCL-2), human fibrosarcoma cells (HT-1080, ATCC: CCL-121) and immortalized human mesenchymal stem cells [53] ) were cultivated in DMEM (Invitrogen, Basel, Switzerland) supplemented with 1% (v/v) penicillin/streptomycin solution (Sigma-Aldrich, Munich, Germany). Wild-type Chinese hamster ovary cells (CHO-K1, ATCC: CCL-61) were cultured in ChoMaster HTS (Cell Culture Technologies GmbH, Gravesano, Switzerland) containing 1% penicillin/streptomycin. All cell types were cultivated at 37 °C in a humidified atmosphere containing 5% CO 2 . For (co-)transfection of BHK-21, CHO-K1, COS-7, HeLa, HT-1080 and human mesenchymal stem cellss, 40,000 cells seeded per well of a 24-well plate 12 h beforetransfection were incubated for 6 h with a 4:1 PEI:DNA mixture (Polyethyleneimine; MW 40,000, Polysciences, Inc., Warrington, USA). After transfection, all cells were cultivated in their specific media containing different inducer concentrations and reporter protein levels were profiled after 48 h unless stated otherwise. For cotransfection of circuit components (pKR135 and pKR153) into HT-1080, a typical transfection efficiency of 61% was reached ( Supplementary Fig. S5 ). SEAP production Production levels of the human placental SEAP were quantified in cell culture supernatants using a p -nitrophenylphosphate-based light-absorbance time course [54] . One hundred microlitres of cell-culture supernatant were heat inactivated for 30 min at 65 °C and centrifuged for 2 min at 14,000 g to remove cell debris. Eighty microlitres of the sample were transferred into a well of a 96-well plate and adjusted to 37 °C. One hundred microlitres of 2 × SEAP buffer (20 mM homoarginine, 1 mM MgCl 2 , 21% (v/v) diethanolamine, pH 9.8) were mixed with 20 μl substrate solution (120 mM para -nitrophenyl phosphate), adjusted to 37 °C and added to the well containing the heat-inactivated sample. The absorbance time course was recorded at 405 nm using an Envision 2104 multilabel plate reader (Perkin Elmer, Waltham, USA). SEAP concentrations in blood samples were quantified using a chemiluminescence-based assay (Roche Diagnostics GmbH, Mannheim, Germany). In brief, 50 μl of heat-inactivated serum (30 min, 65 °C), centrifuged for 30 s at 14,000 g , were transferred to a well of a 96-well plate containing 50 μl inactivation buffer and incubated for 10 min at 22 °C. Next, 50 μl of freshly prepared substrate reagent (50 μl CSPD [3-(4-methoxyspiro[1,2-dioxetane-3,2′(5′-chloro)-tricyclo(3.3.1.1 [3] , [7] decane]-4-yl)phenyl phosphate] mixed with 950 μl substrate buffer) was added to each well and incubated for 10 min at 22 °C before light emission was recored at 477 nm using the Envision 2104 multilabel plate reader (Perkin Elmer). Flow cytometry pDSRed-N1- or pKR135/pKR153-(co)-transfected HT-1080 cell populations were diluted in 1% BSA (Sigma-Aldrich)-containing PBS (137 mM NaCl, 2.7 mM KCl, 4.3 mM Na 2 HPO 4 , 1.4 mM KH 2 PO 4 , pH 7.4; 1 × 10 6 cells per ml) and analysed using a LSRII Fortessa flow cytometer (Becton Dickinson, Allschwil, Switzerland) equipped for DsRed (561 nm laser excitation and 586/15 emission filter) detection and set to exclude dead cells and cell doublets. At least 10,000 cells were recorded per data set and analysed using FACSDiva (BD Biosciences, Franklin Lakes, NJ, USA, version no. 6.1.3.). Blood fat levels Blood cholesterol levels were profiled using a total cholesterol assay kit (Fluoro Cholesterol; Cell Technology, Mountain View, USA). In brief, 50 μl of appropriately ddH 2 O-diluted serum was added per well of a clear-bottom black 96-well plate containing 50 μl of freshly prepared reaction cocktail (20 μl resuspended enzyme mix, 20 μl resuspended cholesterol probe and 960 μl reaction buffer). The plate was incubated in the dark for 1 h at 22 °C and fluorescence was quantified at excitation 530 nm and emission 585 nm using the Envision 2104 multilabel plate reader (Perkin Elmer). Blood phospholipid levels were quantified using a phospholipid assay kit (Abnova GmbH, Heidelberg, Germany). In brief, 20 μl of appropriately Triton X-100 (Sigma-Aldrich)-diluted serum was added per well of a clear-bottom black 96-well plate containing 80 μl of freshly prepared working reagent (85 μl assay buffer, 1 μl PLD enzyme, 1 μl Enzyme Mix and 1 μl Dye Reagent). The plate was incubated in the dark for 30 min at 22 °C and fluorescence was quantified at excitation 530 nm and emission 585 using the Envision 2104 multilabel reader (Perkin Elmer). Pramlintide quantification and activity tests In vitro activity of pramlintide was measured by (co-)transfecting HT-1080 with pKR135/pKR146 or pJWS17 (6 μg DNA, 800,000 cells, 10 cm Petri dish). Forty-eight hours after transfection, the culture medium was transferred to 60,000 HEK-293 cells that had been cotransfected with pCALCR, pRAMP3, pCK53 and pcDNA3.1 at a ratio of 1:1:0.5:7.5 (0.6 μg of total DNA) and SEAP levels were profiled after 48 h. Alternatively, pramlintide was quantified using the human amylin EIA ELISA kit (Phoenix Pharmaceuticals, Burlingame, USA) and pure pramlintide as standard (Feldan, Quebec, Canada). For quantification of pramlintide in mouse serum samples, 96-well plates were coated with 5 μg ml −1 (100 μl per well) rabbit polyclonal anti-human amylin (Amylin H-50, Santa Cruz Biotechnology, Santa Cruz, USA; catalogue number sc-20936, lot. no. I0303; dilution 1:300) in dilution buffer (PBS, 0.5% BSA, 0.01% Tween80, pH 7.4) at 4 °C overnight. Plates were blocked with 200 μl per well PBS/1% BSA, pH 7.4, for 1 h at 22 °C. Pramlintide standard (1–500 μg ml −1 ) and samples (100 μl per well) were diluted (PBS, 0.5% BSA, 0.01% Tween80, pH 7.4) and incubated for 1.5 h at 22 °C. Plates were washed three times with 250 μl per well PBS containing 0.15% Tween-20 and then incubated with 100 μl per well of a mouse monoclonal anti-Amylin (Abcam, Cambridge, UK; catalogue number ab115766, lot no. GR81110-2; dilution 1:450) for 1 h at 22 °C. After three washing steps (250 μl PBS/0.15% Tween-20), the plates were incubated with an anti-mouse horseradish peroxidase-conjugated IgG (GE Healthcare, Buckinghamshire, UK, catalogue number NA931V, lot no. 399402; dilution 1:1,000) for 1 h at 22 °C, washed again (250 μl PBS/0.15% Tween-20) and bound pramlintide was visualized by incubation of the samples with 100 μl per well of 3,3′,5,5′-tetramethylbenzidine substrate (Interchim, Montluçon, France) at 22 °C for 6 min. Reactions were stopped by addition of 2 M sulphuric acid (100 μl per well) and pramlintide was quantified at 450 nm using Envision 2104 multilabel reader (Perkin Elmer). Co-immunoprecipitation Six micrograms of Protein A Dynabeads (Invitrogen Dynal AS, Oslo, Norway) were washed twice with 300 μl co-immunoprecipitation (CoIP) buffer (50 mM Tris, pH 8, 150 mM NaCl, 1 mM EDTA, 1% Triton X-100) containing 6 μl protease inhibitor cocktail (Roche Diagnostics GmbH, Basel, Switzerland) and incubated with 6 μg of the rabbit polyclonal anti-HA antibody (Y-11; Santa Cruz Biotechnology Inc; catalogue number sc-805, lot no. G1210; dilution 1:3) for 4 h while mixing at room temperature on an end-over rotator. pKR151/pMG10-cotransfected HT-1080 cells (1.2 × 10 8 ) were washed twice with 30 ml cold PBS and the cell nuclei were extracted with 45 ml nuclear isolation buffer (300 mM sucrose, 10 mM Tris, pH 8, 5 mM MgCl 2 and 0.5% Triton X-100, 0.1% protease mix) for 10 min at 4 °C. Isolated cell nuclei were resuspended in 2 ml CoIP buffer containing 200 μl protease inhibitor cocktail (Roche Diagnostics GmbH) and 1 μl ml −1 Benzonase (Invitrogen) and sonicated for 15 min and 30 s at 4 °C (320 W, Biorupter Plus, Diagenode S.A, Liège, Belgium). Two millilitres of the resulting nuclear extract was incubated overnight at 4 °C with 30 μl of anti-HA antibody-linked Protein A Dynabeads while mixing on an end-over rotator. The immunocomplexes were washed three times with 500 μl CoIP buffer for 10 min and the immunoprecipitated protein complexes were then visualized by western blot analysis. Western blotting Twenty microlitres of the immunoprecipitated protein complexes were mixed with 5 μl of NuPAGE LSD sample buffer (4 × ; Invitrogen) and 1 μl of 1 M dithiothreitol, resolved on a 4–12% Bis-Tris gel (NuPAGE; Invitrogen) or a 3–8% Tris-Acetate Gel (NuPAGE Novex; Invitrogen) and electroblotted (Trans-Blot SD, Bio-Rad, Reinach, Switzerland) onto an Amersham Hybond-ECL membrane (GE Healthcare, Glattbrugg, Switzerland). The membrane was blocked with 5% (w/v) non-fat dried milk (AppliChem GmbH, Darmstadt, Germany) diluted in PBST (PBS, 0.1% Tween-20) for 30 min at 22 °C and incubated overnight at 4 °C with recommended dilutions of the following primary antibodies: mouse monoclonal anti-GPS2 antibody (Abcam; catalogue number ab53406, lot no. GR61606-3; dilution 1:500), goat polyclonal anti-NCoR antibody (C-20; Santa Cruz Biotechnology Inc.; catalogue number sc-1609, lot no. A2813; dilution 1:200), goat polyclonal anti-HDAC3 antibody (N-19; Santa Cruz Biotechnology Inc.; catalogue number sc-8138, lot no. C1913; dilution 1:200) and goat polyclonal anti-HA antibody (F-7; Santa Cruz Biotechnology Inc.; catalogue number sc-7392, lot no. C081; dilution 1:1,000). The membrane was then washed three times in PBST and incubated for 1 h with a horseradish peroxidase-coupled sheep anti-mouse IgG (GE Healthcare; catalogue number NA931V, lot no. 399402; dilution 1:1,000) or rabbit anti-goat IgG (Sigma-Aldrich; catalogue number A5420, lot no. 043M4763; dilution 1:2,000). The super signal West Femto Western blot detection reagent (Thermo Scientific, Rockford, USA) and the X-ray apparatus Konika Minolta SRX-101A (Konika Minolta GmbH, Langenhagen, Germany) were used for detection. Cytokine measurements TNF-α and IL-6 levels were profiled in the blood of treated animals using murine TNF-α- and IL-6-specific ELISA assays (PeproTech, Rocky Hill, NJ, USA, catalogue numbers 900-M54 (TNF-α) and 900-M50 (IL-6)) according to the manufacturer’s instructions. Intraperitoneal injections of 1 ml 1% (w/v) thioglycollate in ddH 2 O (Sigma-Aldrich) were used as an inflammation-inducing positive control set-up. Animal experiments Intraperitoneal implants were produced by encapsulating pKR135/pMG10- or pKR135/146-transgenic HT-1080 into coherent alginate-poly-( l -lysine)-alginate beads (400 μm; 200 cells per capsule) using an Inotech Encapsulator Research Unit IE-50R (Buchi Labortechnik AG, Flawil, Switzerland) set to the following parameters: 200 μm nozzle with a vibration frequency of 1,023 Hz and 900 V for bead dispersion, 20 ml syringe operated at a flow rate of 403 units. Four hundred microlitres of serum-free DMEM containing 2 × 10 6 microencapsulated transgenic cells (pKR135/pMG10- or pKR135/pKR146-transgenic HT-1080; 200 cells per capsule) were injected intraperitoneally into 14-week-old female CD1 (normal 5 kcal% fat diet; Janvier S.A.S., Le Genest-Saint-Isle, France) or 14-week-old diet-induced obese mice (C57BL/6J, The Jackson Laboratory, Maine, USA) that were on a 10-kcal% (D12450Bi, Research Diets, Inc., NJ) or a 60-kcal% fat diet (D12492i, Research Diets, New Brunswick, USA). CD1 mice implanted with pKR135/pMG10-transgenic HT-1080 received twice daily injections of linoleic or palmitic acid (200 μl, 0-200 mg kg −1 ; linoleic acid, Thermo Fisher Scientific, Geel, Belgium; palmitic acid: Sigma-Aldrich) or oral doses of rapeseed oil (100 and 200 μl; Naturaplan Rapsöl, Coop, Basel, Switzerland). Control mice were treated with capsules containing non-engineered parental HT-1080. Every day, the food intake and body weight of the animals was profiled. After a starvation period of 4 h, blood samples were collected and the serum was isolated using microtainer SST tubes according to the manufacturer’s protocol (Beckton Dickinson, Plymouth, UK) before serum SEAP, blood fat and pramlintide levels were scored as described above. All experiments involving animals were performed according to the directives of the European Community Council (2010/63/EU), approved by the French Republic (no. 69266309), and carried out by Ghislaine Charpin-El Hamri at the Institut Universitaire de Technology, IUTA, F-69622 Villeurbanne Cedex, France. How to cite this article: Rössger, K. et al. A closed-loop synthetic gene circuit for the treatment of diet-induced obesity in mice. Nat. Commun. 4:2825 doi: 10.1038/ncomms3825 (2013).